A peptide derived from laminin-γ3 reversibly impairs spermatogenesis in rats Cellular events that occur across the seminiferous epithelium in the mammalian testis during spermatogenesis are tightly coordinated by biologically active peptides released from laminin chains. Laminin-γ3 domain IV is released at the apical ectoplasmic specialization during spermiation and mediates restructuring of the blood–testis barrier, which facilitates the transit of preleptotene spermatocytes. Here we determine the biologically active domain in laminin-γ3 domain IV, which we designate F5 peptide, and show that the overexpression of this domain, or the use of a synthetic F5 peptide, in Sertoli cells with an established functional blood–testis barrier reversibly perturbs blood–testis barrier integrity in vitro and in the rat testis in vivo. This effect is mediated via changes in protein distribution at the Sertoli and Sertoli–germ–cell cell interface and by phosphorylation of focal adhesion kinase at Tyr 407 . The consequences are perturbed organization of actin filaments in Sertoli cells, disruption of the blood–testis barrier and spermatid loss. The impairment of spermatogenesis suggests that this laminin peptide fragment may serve as a contraceptive in male rats. During the seminiferous epithelial cycle of spermatogenesis in the mammalian testis, multiple cellular events take place across the seminiferous epithelium, which include spermatogonial self-renewal via mitosis, meiosis, spermiogenesis and spermiation, which are supported by Sertoli cells [1] , [2] , [3] , [4] , [5] , [6] , [7] , [8] , [9] . Although these cellular events are tightly coordinated and regulated, the underlying regulatory mechanisms remain unknown. A recent report has shown that fragments of laminin-β3 and -γ3 chains that are expressed by elongating/elongated spermatids and are components of the α6β1-integrin/laminin-α3β3γ3 adhesion protein complex at the apical ectoplasmic specialization (ES) [10] , [11] , a testis-specific actin-based adherens junction [12] , [13] , are likely generated at spermiation via the action of metalloprotease-2 [14] as the result of apical ES disruption/degeneration at the luminal edge of the tubule acting as biologically active, autocrine peptides to induce blood–testis barrier (BTB) restructuring to facilitate the transit of preleptotene spermatocytes across the BTB [15] . In short, these two cellular events, namely spermiation and BTB restructuring, which occur at the opposite ends of the seminiferous epithelium, are coordinated by biologically active laminin fragments. This observation prompted us to hypothesize the presence of an apical ES–BTB functional axis [15] , which coordinates cellular events that occur at different cellular compartments in the seminiferous epithelium [12] . Studies from other epithelia have also demonstrated that laminin fragments are biologically active, capable of altering cellular function, including cell movement and cell adhesion [13] , [16] , [17] , [18] , [19] . In addition, the concept of an apical ES–BTB functional axis is supported by recent studies using the phthalate-induced Sertoli cell injury model [20] , [21] , [22] . Moreover, we have recently shown that activated FAK, p-FAK-Tyr 407 , appears to be a crucial signalling molecule that serves as a ‘molecular switch’ in this axis via its restrictive spatiotemporal expression at the apical ES and the BTB to regulate this functional axis [23] . We report herein the identification of the biologically active domain residing in the laminin-γ3 chain. Overexpression of this domain in Sertoli cells was found to perturb the Sertoli cell tight junction (TJ)-barrier function in vitro , and the use of a synthetic peptide based on this domain also perturbed BTB function reversibly both in vitro and in vivo . The peptide induced germ cell loss from the testis, thereby impairing spermatogenesis. We also identified a mechanism by which this peptide might exert its effects, which involves phosphorylation of FAK-Tyr 407 . Laminin fragments regulate Sertoli cell TJ function Studies in vitro were performed with a Sertoli cell culture system by using primary Sertoli cells with negligible Leydig and germ cell contamination as earlier described [24] , which also formed a functional TJ-permeability barrier with ultrastructures of TJ, basal ES, gap junction and desmosome when examined under electron microscopy [25] , [26] , [27] that mimicked the BTB in vivo [2] . This system is widely used by investigators in the field to study BTB function and its regulation [30] . In short, DNA constructs corresponding to the entire or portions of domain IV of the laminin-γ3 chain were cloned into the pCIneo mammalian expression vector ( Fig. 1a–c ), which were used to transfect Sertoli cells that had been cultured alone for 3 days ( Fig. 1d ) with an established functional TJ-permeability barrier ( Fig. 1 e ) with a transfection efficiency of ~15–20% (see Supplementary Methods ). As Sertoli cells do not express laminin-γ3 chain nor its fragments because laminin-γ3 is a spermatid protein at the apical ES in the rat testis [10] , [15] , expression of laminin-γ3 DIV and the corresponding fragments F1–F5 in these Sertoli cell cultures ( Fig. 1d ) thus illustrate transient overexpression of these genes when cells were harvested 48 h after transfection for RT-PCR using primers specific to these genes ( Supplementary Table S1 ). It was noted that besides laminin-γ3 DIV, which was earlier shown to be biologically active and to disrupt Sertoli cell TJ-barrier function [15] , only F2 and F5 were capable of perturbing the Sertoli cell BTB function, but the F5 fragment was more potent in perturbing the TJ-barrier ( Fig. 1e ), illustrating the biologically active domain is residing in F5, perhaps also in part in F2 (see Fig. 1b ). Attempts were made to further define the biologically active domain residing in the overlapping F2 and F5 fragments by preparing three additional cDNA constructs designated F6, F7 and F8 (see Supplementary Fig. S1 ); however, overexpression of these constructs in Sertoli cells showed that they were biologically inactive, incapable of perturbing the Sertoli cell TJ-barrier function or of reducing the expression of TJ- (for example, occludin) and/or basal ES- (for example, N-cadherin, β-catenin) proteins at the Sertoli cell BTB ( Supplementary Fig. S1a–e ), indicating stretches of sequences in these two overlapping fragments are crucial to confer biological activity and to perturb the Sertoli cell TJ-barrier. 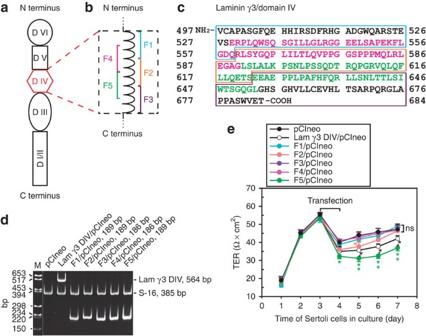Figure 1: Preparation of laminin-γ3 domain IV cDNA constructs to assess their biological activity. (a) Schematic drawing illustrating different functional domains of laminin-γ3 chain. Laminin-γ3 domain IV (DIV, in red) was selected based on earlier studies that this domain is biologically active in regulating BTB dynamics15, and it was further divided into five fragments of F1–F5 as shown inbto assess their effects on BTB function. (c) cDNA-deduced amino-acid sequence of laminin-γ3 DIV (GenBank accession codeXM_231139) is shown, illustrating the sequences of F1 (blue boxed area), F2 (orange boxed area), F3 (purple boxed area), F4 (pink coloured text) and F5 (green coloured text). (d) RT-PCR illustrating the expression of laminin-γ3 DIV and the five different fragments (seea) in Sertoli cells after transfection with corresponding vectors versus pCIneo alone for 3 days. Cells transfected with pCIneo alone served as a negative control since Sertoli cellsper sedid not express laminin-γ3 chains, which are exclusively expressed by elongating/elongated spermatids10. S-16 served as an internal PCR control. Identity of the PCR product was confirmed by direct nucleotide sequencing at GeneWiz Inc (South Plainfield, NJ). M, DNA markers; bp, base-pair. (e) Changes in the Sertoli cell TJ-permeability barrier function following transient expression of different fragments of laminin-γ3 DIV versus DIV (positive control) and pCIneo alone (negative control) on day 3 for 24 h by quantifying transepithelial electrical resistance (TER) across the Sertoli cell epithelium in bicameral units (n=3). This experiment was repeated three times using different batches of Sertoli cells which yielded similar results. *P<0.05; **P<0.01. Figure 1: Preparation of laminin-γ3 domain IV cDNA constructs to assess their biological activity. ( a ) Schematic drawing illustrating different functional domains of laminin-γ3 chain. Laminin-γ3 domain IV (DIV, in red) was selected based on earlier studies that this domain is biologically active in regulating BTB dynamics [15] , and it was further divided into five fragments of F1–F5 as shown in b to assess their effects on BTB function. ( c ) cDNA-deduced amino-acid sequence of laminin-γ3 DIV (GenBank accession code XM_231139 ) is shown, illustrating the sequences of F1 (blue boxed area), F2 (orange boxed area), F3 (purple boxed area), F4 (pink coloured text) and F5 (green coloured text). ( d ) RT-PCR illustrating the expression of laminin-γ3 DIV and the five different fragments (see a ) in Sertoli cells after transfection with corresponding vectors versus pCIneo alone for 3 days. Cells transfected with pCIneo alone served as a negative control since Sertoli cells per se did not express laminin-γ3 chains, which are exclusively expressed by elongating/elongated spermatids [10] . S-16 served as an internal PCR control. Identity of the PCR product was confirmed by direct nucleotide sequencing at GeneWiz Inc (South Plainfield, NJ). M, DNA markers; bp, base-pair. ( e ) Changes in the Sertoli cell TJ-permeability barrier function following transient expression of different fragments of laminin-γ3 DIV versus DIV (positive control) and pCIneo alone (negative control) on day 3 for 24 h by quantifying transepithelial electrical resistance (TER) across the Sertoli cell epithelium in bicameral units ( n =3). This experiment was repeated three times using different batches of Sertoli cells which yielded similar results. * P <0.05; ** P <0.01. Full size image Laminin- γ 3 fragments regulate protein expression at the BTB The biological effects of F2 and F5 fragments and the laminin-γ3 DIV versus control and other non-active fragments as noted in Fig. 1 were further assessed by their ability to modulate the steady-state levels of TJ- (for example, occludin, JAM-A), TJ-regulatory- (for example, FAK, p-FAK-Tyr 407 ) and basal ES- (for example, N-cadherin, β-catenin) proteins at the Sertoli cell BTB on day 3 after transfection (that is, day 6 after cell plating) ( Fig. 2a ). The steady-state protein levels of occludin, JAM-A and p-FAK-Tyr 407 , but not FAK, N-cadherin and β-catenin were found to be significantly reduced in Sertoli cell epithelium following overexpression of F5 peptide and laminin-γ3 DIV ( Fig. 3a ). The finding that the expression of p-FAK-Tyr 407 was downregulated by these fragments was significant as p-FAK-Tyr 407 is a crucial BTB regulatory protein [23] . F2 fragment was also active, but its biological effect in disrupting Sertoli cell BTB protein expression was considerably lower versus F5 ( Fig. 2a ), consistent with data shown in Fig. 1e . Similarly, F6, F7 and F8 also had no apparent effects in perturbing the steady-state level of occludin in the Sertoli cell epithelium ( Supplementary Fig. S1e ). 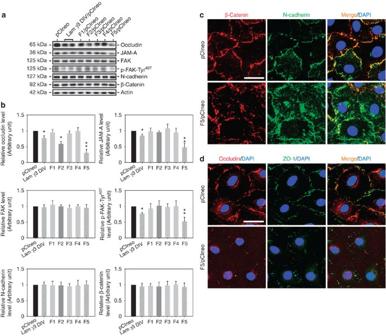Figure 2: Laminin-γ3 fragments affect protein expression and localization at the Sertoli cell BTB. (a) On day 3, Sertoli cells with a functional BTB were transfected with different expression vectors for 24 h and terminated 48 h thereafter for immunoblotting, illustrating changes in the levels of integral membrane proteins (for example, occludin, JAM-A, N-cadherin), adaptor protein (for example, β-catenin) and regulatory proteins (for example, FAK, p-FAK-Tyr407). (b) Bar graphs summarize results shown ina. Each bar is a mean±s.d. ofn=5 experiments, and data were normalized against actin. The protein levels in cells transfected with pCIneo alone were arbitrarily set at 1, against which one-way analysis of variance and Dunnett’s test were performed. *P<0.05; **P<0.01. (c) Overexpression of F5 peptide in Sertoli cells caused considerable re-distribution of basal ES proteins at the BTB: β-catenin (red) and N-cadherin (green) at the Sertoli cell–cell interface, moving away from cell surface and into cell cytosol on day 3 after transfection. Overexpression of F5 peptide also changed localization and/or distribution of TJ proteins at the BTB: occludin (red) and ZO-1 (green) at the Sertoli cell–cell interface. Co-localized proteins appeared as ‘orange’ in merged images. Nuclei were visualized by 4',6-diamidino-2-phenylindole (DAPI) (blue). Scale bar=10 μm incandd, which applies to all images in both panels. Figure 2: Laminin-γ3 fragments affect protein expression and localization at the Sertoli cell BTB. ( a ) On day 3, Sertoli cells with a functional BTB were transfected with different expression vectors for 24 h and terminated 48 h thereafter for immunoblotting, illustrating changes in the levels of integral membrane proteins (for example, occludin, JAM-A, N-cadherin), adaptor protein (for example, β-catenin) and regulatory proteins (for example, FAK, p-FAK-Tyr 407 ). ( b ) Bar graphs summarize results shown in a . Each bar is a mean±s.d. of n =5 experiments, and data were normalized against actin. The protein levels in cells transfected with pCIneo alone were arbitrarily set at 1, against which one-way analysis of variance and Dunnett’s test were performed. * P <0.05; ** P <0.01. ( c ) Overexpression of F5 peptide in Sertoli cells caused considerable re-distribution of basal ES proteins at the BTB: β-catenin (red) and N-cadherin (green) at the Sertoli cell–cell interface, moving away from cell surface and into cell cytosol on day 3 after transfection. Overexpression of F5 peptide also changed localization and/or distribution of TJ proteins at the BTB: occludin (red) and ZO-1 (green) at the Sertoli cell–cell interface. Co-localized proteins appeared as ‘orange’ in merged images. Nuclei were visualized by 4',6-diamidino-2-phenylindole (DAPI) (blue). Scale bar=10 μm in c and d , which applies to all images in both panels. 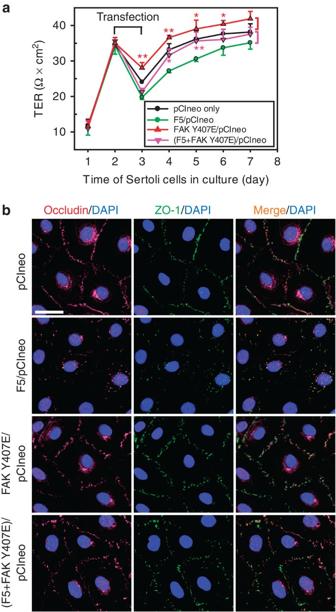Figure 3: Laminin F5 peptide perturbs Sertoli cell TJ function via p-FAK-Tyr407. (a) To examine the mechanism by which the F5 peptide perturbs the Sertoli cell TJ-permeability barrier function as shown inFigs 1and2, p-FAK-Tyr407, a molecular ‘switch’ in the apical ES–BTB axis to regulate BTB restructuring and apical ES adhesion23, was expressed either alone as a phosphomimetic mutant (FAK Y407E/pCIneo) or co-expressed with F5 [(F5+FAK Y407E)/pCIneo]. Co-expression of FAK phosphomimetic mutant FAK Y407E with F5-peptide in Sertoli cells blocked the F5-induced TJ-barrier disruption, which is likely mediated by the ability of p-FAK-Tyr407to promote the distribution of occludin and ZO-1 at the Sertoli cell–cell interface shown inb, thereby stabilizing the Sertoli TJ barrier. Each data point inais a mean±s.d. ofn=4 of a representative experiment, and this experiment and data shown inbwere repeated three times, which yielded similar results. *P<0.05; **P<0.01. Scale bar=10 μm, which applies to all remaining micrographs. Full size image Figure 3: Laminin F5 peptide perturbs Sertoli cell TJ function via p-FAK-Tyr 407 . ( a ) To examine the mechanism by which the F5 peptide perturbs the Sertoli cell TJ-permeability barrier function as shown in Figs 1 and 2 , p-FAK-Tyr 407 , a molecular ‘switch’ in the apical ES–BTB axis to regulate BTB restructuring and apical ES adhesion [23] , was expressed either alone as a phosphomimetic mutant (FAK Y407E/pCIneo) or co-expressed with F5 [(F5+FAK Y407E)/pCIneo]. Co-expression of FAK phosphomimetic mutant FAK Y407E with F5-peptide in Sertoli cells blocked the F5-induced TJ-barrier disruption, which is likely mediated by the ability of p-FAK-Tyr 407 to promote the distribution of occludin and ZO-1 at the Sertoli cell–cell interface shown in b , thereby stabilizing the Sertoli TJ barrier. Each data point in a is a mean±s.d. of n =4 of a representative experiment, and this experiment and data shown in b were repeated three times, which yielded similar results. * P <0.05; ** P <0.01. Scale bar=10 μm, which applies to all remaining micrographs. Full size image Overexpression of F5 fragment affects protein distribution Sertoli cells cultured alone for 3 days with an established TJ-permeability barrier were transfected with F5/pCIneo plasmid DNA versus pCIneo vector alone (control). Twenty-four hours thereafter, transfection mixture was removed and cells were cultured for an additional 2 days before being subjected to dual-labeled immunofluorescence analysis using corresponding antibodies (see Supplementary Table S2 ). In control cells, basal ES proteins N-cadherin (green) and β-catenin (red), and TJ proteins occludin (red) and ZO-1 (green) were co-localized mostly at the Sertoli cell–cell interface ( Fig. 2c ). In cells transfected with the F5 fragment, the localization of both N-cadherin and β-catenin became disorganized, as both proteins seemed to move away from the cell surface and into cell cytosol ( Fig. 2c ). However, we found a considerable loss of occludin and ZO-1 at the Sertoli cell–cell interface ( Fig. 2d ), consistent with a reduction in the steady-state level of occludin in these cells (see Fig. 2d ). Overexpression of F5 peptide fragment also caused a loss in the co-localization of adhesion protein complexes N-cadherin/β-catenin and occludin/ZO-1 ( Fig. 2c ). These findings ( Fig. 2 ) support results shown in Fig. 1e , illustrating that the disruption of the Sertoli cell TJ-barrier following F5 peptide overexpression in Sertoli cells is mediated by changes in protein distribution at the Sertoli cell–cell interface. FAK Y407E blocks F5 peptide-induced TJ disruption Phosphorylation of FAK at Tyr 407 (p-FAK-Tyr 407 ) is known to regulate BTB dynamics by increasing the tightness of the Sertoli cell TJ-permeability barrier [23] . As shown in Fig. 2a , overexpression of the F5 fragment in Sertoli cells that perturbed the TJ-barrier function (see Fig. 1e ) downregulated the expression of p-FAK-Tyr 407 . Overexpression of a phosphomimetic mutant FAK Y407E, however, promoted the Sertoli cell TJ-barrier, making it ‘tighter’, and its co-expression with F5 fragment (F5/pCIneo) was capable of blocking the F5-induced TJ-barrier disruption ( Fig. 3a ), illustrating p-FAK-Tyr 407 is a crucial signalling molecule downstream of the biologically active laminin fragment in the apical ES–BTB axis. Studies by dual-labeled immunofluorescence analysis also demonstrated that co-expression of FAK Y407E mutant prevented the F5 fragment-mediated mis-distribution of occludin and ZO-1 at the Sertoli cell–cell interface ( Fig. 3b ), thereby illustrating p-FAK-Tyr 407 is an important signalling partner of the laminin fragment in regulating the apical ES–BTB axis. F5 peptide perturbs Sertoli cell TJ function in vitro We next added a synthetic peptide corresponding to the first 50 amino acids of F5 fragment designated F5 peptide ( Fig. 4a ) to Sertoli cells cultured on bicameral units on day 3 when a functional TJ-barrier was established ( Fig. 4b ). We found that the presence of the synthetic F5 peptide perturbed the Sertoli cell TJ-barrier ( Fig. 4b ). This disruptive effect was reversible, as its removal by washing Sertoli cells with F12/DMEM without the synthetic peptide allowed the disrupted TJ-barrier to be ‘resealed’ ( Fig. 4b ). However, the 22-amino acid myotubularin-related protein 2 (MTMR2) had no apparent effects on the TJ-barrier, similar to the PBS control ( Fig. 4b ), consistent with an earlier report [31] . 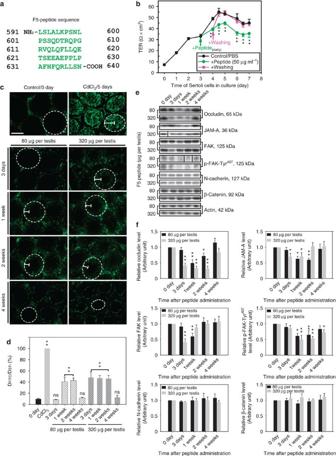Figure 4: Laminin F5 peptide reversibly perturbs BTB functionin vitroand in vitro. (a) Amino-acid residues (green) of the synthetic F5-peptide based on laminin-γ3 DIV. Numerals in ‘black’ denote the sequence of laminin-γ3 chain (seeFig. 1a–c). (b) Effects of the synthetic F5-peptide on the Sertoli cell TJ-permeability barrier. Peptide at 50 μg ml−1(~10 μM) was added on day 3 (‘green’ arrow), which was either included in the daily replacement medium (‘green’) (n=3) or removed by washing on day 4 (‘pink’ arrow) in medium without peptide (‘pink’) versus PBS control. When F5 peptide was removed, the disrupted TJ barrier was ‘resealed’, illustrating the disruptive effect was reversible. Each data point is a mean±s.d. ofn=3 of a representative experiment, and this experiment was repeated three times which yielded similar results. **P<0.01. (c) BTB integrity assay was performed to assess the ability of an intact BTB to block the movement of FITC-inulin across the BTB from the basal compartment near the basement membrane (annotated by ‘white’ dotted line) to the adluminal compartment. Results of the BTB integrity assay are shown in normal testes (control) versus rats treated with CdCl2and different peptide treatment groups: 80 μg per testis (or ~10 μM) and 320 μg per testis (~40 μM). Scale bar=150 μm inc, which also applies to all remaining micrographs. (d) Histograms summarizing the data based on findings shown incby comparing the distance of FITC-inulin diffused into the epithelium (DFITC) (annotated by the ‘white bracket’) versus the radius of a seminiferous tubule (DSTr) (average of the longest and shortest axes for sections of oval-shaped tubules) (n=200 tubules from testes of three rats in each group). **P<0.01; ns, not significantly different. (e) Immunoblot analysis of different target proteins at the BTB in adult rat testes at different time points after peptide administration. (f) Histograms summarizing data shown inewithn=3 rats for each time point. *P<0.05; **P<0.01. Figure 4: Laminin F5 peptide reversibly perturbs BTB function in vitro and in vitro. ( a ) Amino-acid residues (green) of the synthetic F5-peptide based on laminin-γ3 DIV. Numerals in ‘black’ denote the sequence of laminin-γ3 chain (see Fig. 1a–c ). ( b ) Effects of the synthetic F5-peptide on the Sertoli cell TJ-permeability barrier. Peptide at 50 μg ml −1 (~10 μM) was added on day 3 (‘green’ arrow), which was either included in the daily replacement medium (‘green’) ( n =3) or removed by washing on day 4 (‘pink’ arrow) in medium without peptide (‘pink’) versus PBS control. When F5 peptide was removed, the disrupted TJ barrier was ‘resealed’, illustrating the disruptive effect was reversible. Each data point is a mean±s.d. of n =3 of a representative experiment, and this experiment was repeated three times which yielded similar results. ** P <0.01. ( c ) BTB integrity assay was performed to assess the ability of an intact BTB to block the movement of FITC-inulin across the BTB from the basal compartment near the basement membrane (annotated by ‘white’ dotted line) to the adluminal compartment. Results of the BTB integrity assay are shown in normal testes (control) versus rats treated with CdCl 2 and different peptide treatment groups: 80 μg per testis (or ~10 μM) and 320 μg per testis (~40 μM). Scale bar=150 μm in c , which also applies to all remaining micrographs. ( d ) Histograms summarizing the data based on findings shown in c by comparing the distance of FITC-inulin diffused into the epithelium ( D FITC ) (annotated by the ‘white bracket’) versus the radius of a seminiferous tubule ( D STr ) (average of the longest and shortest axes for sections of oval-shaped tubules) ( n =200 tubules from testes of three rats in each group). ** P <0.01; ns, not significantly different. ( e ) Immunoblot analysis of different target proteins at the BTB in adult rat testes at different time points after peptide administration. ( f ) Histograms summarizing data shown in e with n =3 rats for each time point. * P <0.05; ** P <0.01. Full size image F5 peptide reversibly disrupts BTB integrity in vivo To validate whether the findings shown in Fig. 4a are physiologically relevant, we sought to examine the effects of the synthetic F5 peptide on the BTB integrity in vivo by treating rats with increasing doses of the synthetic F5 peptide via intratesticular injection. In control rat testes ( Fig. 4c ), administration of fluorescein isothiocyanate (FITC)-inulin (green fluorescence) to rats at the jugular vein was found to be excluded from entering the adluminal compartment of the epithelium, consistent with the presence of a functional BTB located near the basement membrane ( Fig. 4c ). However, when rats were treated with CdCl 2 , which perturbs BTB integrity [32] , [33] , [34] , a FITC signal was readily detected in the entire seminiferous epithelium beyond the BTB, including the tubule lumen by day 5 ( Fig. 4c ). However, in rats treated with the F5 peptide at doses of 80 μg per testis (low-dose, ~10 μM) or 320 (high-dose, ~40 μM), BTB integrity was compromised dose-dependently over the next 4 weeks ( Fig. 4c ), even though this damage was not as severe as the CdCl 2 -induced irreversible BTB disruption. More importantly, the disrupted BTB induced by the synthetic F5 peptide was ‘resealed’ after 4 weeks in both the low- and high-dose groups ( Fig. 4c ). Findings shown in Fig. 4c were further analysed semi-quantitatively by comparing the distance travelled by FITC-inulin beyond the BTB near the basement membrane ( D FITC ) versus the radius of the seminiferous tubule ( D STr ) ( Fig. 4d ). These findings also confirm results shown in Figs 1e and 2c and Fig. 4b . When lysates from these rat testes were used for immunoblot analysis to quantify changes in the steady-state levels of TJ (for example, occludin, JAM-A), TJ-regulatory (for example, FAK and p-FAK-Tyr 407 ) and basal ES (for example, N-cadherin, β-catenin) proteins, a dose-dependent downregulation on the expression of the TJ- and TJ-regulatory proteins, but not the basal ES proteins, was noted ( Fig. 4e ). For instance, a transient downregulation of p-FAK-Tyr 407 was noted ( Fig. 4e ), consistent with findings in vitro shown in Fig. 2a ). Synthetic F5 peptide impairs spermatogenesis in rats To test whether local administration of the peptide that perturbed the BTB in vivo would affect the status of spermatogenesis in the seminiferous epithelium, synthetic F5 peptide at doses of 80 μg per testis (low-dose, 10 μM) or 320 μg per testis (high-dose, 40 μM) was administered via intratesticular injection, and histological analysis was performed following hematoxylin and eosin staining using cross-sections of paraffin-embedded testes ( Fig. 5a–e ). Although this treatment did not elicit statistically significant changes in testis weight over the 16-week experiment period as cell adhesion was affected in only ~40% of the tubules examined ( Fig. 5f ), possibly the result of limited access of the F5 peptide to all tubules via local administration, histological analysis of these testes revealed the synthetic F5 peptide caused germ cell depletion from the epithelium, mostly elongated, elongating or round spermatids and some late spermatocytes in treatment versus control groups ( Fig. 5a–g ; Supplementary Fig. S2 ). This disruptive effect on germ cell adhesion was detectable 3 days after treatment in the high-dose group, and the progressive damage in the seminiferous epithelium in both groups was clearly visible ( Fig. 5b–e ) and quantifiable ( Fig. 5f ), illustrating the scope of damage in the epithelium following synthetic F5 peptide administration. For instance, the tubule diameter was reduced by ~40% ( Fig. 5f ) in ~40% of the tubules randomly scored, consistent with the observations shown in Fig. 5a–e . The disruptive effects of the F5 peptide on the status of spermatogenesis were reversible, as spermatogenesis gradually rebounded 16 weeks after treatment in the low-dose group ( Supplementary Fig. S2 ). In a second control group, in which rats were treated with MTMR2 peptide at 50 μM (200 μg peptide/testis) (see Supplementary Methods ), no alterations on the status of spermatogenesis were noted at 1-, 4- and 8-week post treatment, consistent with an earlier report [31] , illustrating the specificity of the F5 peptide in disrupting spermatogenesis. 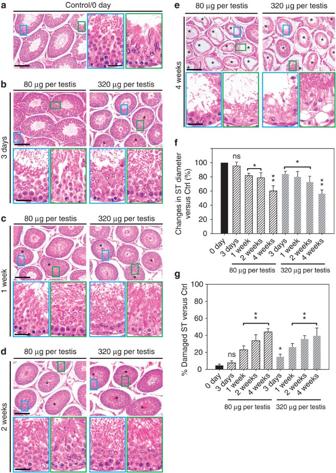Figure 5: Laminin F5 peptide impairs spermatogenesis and induces germ cell loss from the testis. Peptide or vehicle control (0.89% NaCl, seea) was injected into each testis of a group of adult rats (~250–275 g body weight) withn=3 rats per time point in each treatment group versus controls rats were terminated at specified time points at 3 days and 1, 2 or 4 weeks thereafter. (b–e) Representative photographs of paraffin sections of testes stained with hematoxylin and eosin from rats treated with the synthetic F5 peptide at either 80 or 320 μg per testis. Vehicle control is shown ina. Morphometric changes (for example, shrinkage of tubule, and % of damaged seminiferous tubules (ST) manifested by germ cell exfoliation—annotated by asterisks in tubules) of the tubules (n=200 tubules from three rat testes) are summarized in the bar graphs shown infandg. Bar=150 μm ina, and the micrographs on the left panels inb–e, which applies to the micrographs on the right panelsb–e. Bar=50 μm in micrograph encircled in ‘blue’, which applies to all micrographs encircled in ‘blue’ and ‘green’ ina–e. The ‘blue’ and ‘green’ encircled micrographs are magnified images of the corresponding boxed areas of the lower magnification. ns, not significantly different by analysis of variance; *P<0.05; and **P<0.01 when compared with normal control rats at time 0. Ctrl, control. Figure 5: Laminin F5 peptide impairs spermatogenesis and induces germ cell loss from the testis. Peptide or vehicle control (0.89% NaCl, see a ) was injected into each testis of a group of adult rats (~250–275 g body weight) with n =3 rats per time point in each treatment group versus controls rats were terminated at specified time points at 3 days and 1, 2 or 4 weeks thereafter. ( b – e ) Representative photographs of paraffin sections of testes stained with hematoxylin and eosin from rats treated with the synthetic F5 peptide at either 80 or 320 μg per testis. Vehicle control is shown in a . Morphometric changes (for example, shrinkage of tubule, and % of damaged seminiferous tubules (ST) manifested by germ cell exfoliation—annotated by asterisks in tubules) of the tubules ( n =200 tubules from three rat testes) are summarized in the bar graphs shown in f and g . Bar=150 μm in a , and the micrographs on the left panels in b – e , which applies to the micrographs on the right panels b – e . Bar=50 μm in micrograph encircled in ‘blue’, which applies to all micrographs encircled in ‘blue’ and ‘green’ in a – e . The ‘blue’ and ‘green’ encircled micrographs are magnified images of the corresponding boxed areas of the lower magnification. ns, not significantly different by analysis of variance; * P <0.05; and ** P <0.01 when compared with normal control rats at time 0. Ctrl, control. Full size image F5 peptide affects protein localization in the testis Findings shown in Figs 3 , 4 , 5 thus illustrate that the synthetic F5 peptide is capable of inducing BTB disruption and germ cell loss in vivo after its intratesticular administration. We next used immunohistochemistry to assess changes in the localization of TJ proteins, such as occludin, at the BTB in the seminiferous epithelium ( Fig. 6 ). Occludin was selected as a BTB marker protein because this integral membrane protein is abundantly found in the rat testis and its expression is restricted to the BTB [9] . Furthermore, its knockout in mice (occludin −/− ) led to infertility by 36–60 week of age in which tubules were devoid of all spermatocytes and spermatids [35] , [36] (but rats remained fertile by 6- to 10- week of age when other TJ proteins, such as claudin-3 and JAM-A, apparently could supersede and transiently maintain the BTB integrity). In normal (control) rat testes, occludin was detected near the basal compartment of the epithelium, closely localized to the basement membrane, consistent with its localization at the BTB in seminiferous tubules ( Fig. 6 ). However, by 1-week in both the low-and high-dose F5 peptide-treated groups, the expression of occludin was downregulated ( Fig. 6 ), consistent with immunoblotting data shown in Fig. 4e when the BTB was transiently disrupted at this time ( Fig. 4c ). However, by 4-week in both F5 peptide-treated groups, the expression of occludin had rebounded, consistent with immunoblotting data shown in Fig. 4e . Interestingly, it was still found near the basement membrane, but was ‘diffusely’ localized, surrounding the base of the tubule ( Fig. 6 ). In some seminiferous tubules in rats from the low- and more tubules in the high-dose groups by 4-week, occludin was found to be very intensely localized at the BTB in tubules that were completely devoid of germ cells ( Fig. 6 ), analogous to the Sertoli cell-only syndrome. 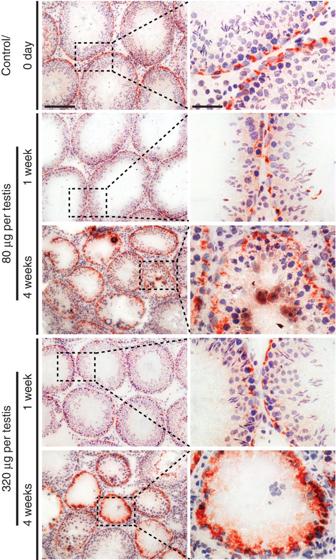Figure 6: Laminin F5 peptide perturbs occludin distribution at the BTB. Normal rat testis (control, 0-day), displaying normal distribution of occludin at the BTB versus rats that received either 80 μg (~10 μM) or 320 μg (~40 μM) F5 peptide per testis by 1 week and 4 weeks with noticeable germ cell loss from the tubules. Micrographs on the right panel are the corresponding magnified images of the boxed area shown on the left panel. Bar=150 μm in the first micrograph on the left panel and scale bar=50 μm in the first micrograph on the right panel, which apply to remaining micrographs in the same panel. Figure 6: Laminin F5 peptide perturbs occludin distribution at the BTB. Normal rat testis (control, 0-day), displaying normal distribution of occludin at the BTB versus rats that received either 80 μg (~10 μM) or 320 μg (~40 μM) F5 peptide per testis by 1 week and 4 weeks with noticeable germ cell loss from the tubules. Micrographs on the right panel are the corresponding magnified images of the boxed area shown on the left panel. Bar=150 μm in the first micrograph on the left panel and scale bar=50 μm in the first micrograph on the right panel, which apply to remaining micrographs in the same panel. Full size image For basal ES proteins N-cadherin and β-catenin at the BTB [12] , [37] , both proteins were found to co-localize at the BTB in control rat testes, forming a ‘belt-like’ ultrastructure surrounding the base of the entire seminiferous tubule ( Supplementary Fig. S3A–E ). However, in testes obtained from rats at 4 weeks in either the low- or the high-dose synthetic F5 peptide-treated group, although these two basal ES proteins remained co-localized at the BTB even when tubules were shrunk by ~40% and the BTB was disrupted (see also Figs 4 and 5 ), both N-cadherin and β-catenin were found to be mis-localized, analogous to occludin shown in Fig. 6 and also data shown in Fig. 2c regarding their mis-localization, as these proteins were no longer confined to the BTB in the seminiferous epithelium, instead, they were mis-localized, associated with apical junctions, and abnormally distributed ( Supplementary Fig. S3 ). F5 peptide exerts its effects via p-FAK-Tyr 407 A recent report has shown that p-FAK-Tyr 407 promotes adhesion at the apical ES and the BTB via its restrictive spatiotemporal expression during the epithelial cycle [23] . During the F5 peptide-induced BTB disruption, a mis-localization of p-FAK-Tyr 407 and its downregulation at the BTB were detected, in which p-FAK-Tyr 407 no longer tightly associated with the BTB, instead it was diffusing away from the site of the BTB in the seminiferous epithelium and its expression was downregulated in some tubules ( Fig. 7a ). Interestingly, the expression of p-FAK-Tyr 407 was almost abolished at the BTB in CdCl 2 -treated rats when the BTB was badly damaged ( Fig. 7c ; Fig. 4c ). Prominent changes in the localization of p-FAK-Tyr 407 at the apical ES were initially detected at 3 days in the F5 peptide-treated rats, where p-FAK-Tyr 407 no longer restricted to the concave side of the elongating spermatid heads. Instead, p-FAK-Tyr 407 was found to engulf both the concave and convex sides of the spermatid heads ( Fig. 7 ). By 1 and 2 weeks, p-FAK-Tyr 407 staining at the apical ES considerably diminished, becoming almost non-detectable in most elongating spermatids and many of these spermatids lost their polarity with their heads pointing randomly to all directions instead of towards the basement membrane (see ‘white’ arrowheads in Fig. 7 ) as seen in control rats. By 4 weeks, virtually no elongating/elongated spermatids were found in the affected tubules; instead, p-FAK-Tyr 407 was found in vesicular structures ( Fig. 7 ), which appeared to be cytoplasmic droplets as reported [23] . These findings thus illustrate that the F5 peptide mediated its effects by downregulating and/or redistributing p-FAK-Tyr 407 in the seminiferous epithelium along the apical ES-BTB axis, which in turn, perturbed cell adhesion at the apical ES and the BTB, leading to germ cell loss ( Fig. 5a , Supplementary Fig. S2 ) and BTB disruption ( Fig. 4 ). 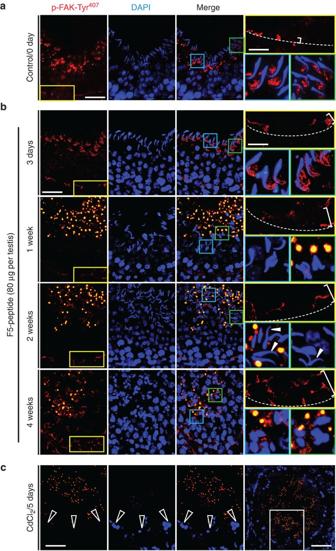Figure 7: Laminin F5-peptide disrupts BTB and spermatid adhesion via p-FAK-Tyr407. Testes received vehicle (control) at time 0 (a) versus synthetic F5-peptide at 80 μg per testis (~10 μM), and terminated at 3 days, and 1, 2 and 4 weeks (b), and positive control where rats were treated with CdCl2(5 mg kg−1body weight, intraperitoneal, for 5 days) (c). In control testes, p-FAK-Tyr407was localized near the basement membrane consistent with its localization at the BTB (see ‘yellow’ boxed area in the micrograph on the left, which was magnified in the right panel (top) in each row with the relative BTB location annotated by the ‘broken white-line’); p-FAK-Tyr407was also found in the adluminal compartment, restricted almost exclusively to the concave side of the spermatid head at the apical ES (see ‘blue’ and ‘green’ boxed areas in the micrograph on the third column, which were magnified in the right panel (bottom) in each row). Following F5 peptide treatment, p-FAK-Tyr407was downregulated and mis-localized at the BTB, as it no longer restricted to the BTB, but diffused away (see ‘white’ bracket on the top right panel of each column in treatment groups versus control rats, which was widened over time in treatment groups). p-FAK-Tyr407was also downregulated and its localization at the apical ES also shifted from the concave to cover the convex side of the spermatid head by 3-day, and p-FAK-Tyr407no longer associated with the apical ES in most elongated spermatids by 1 and 2 weeks, and by 4 weeks as elongated spermatids were not found in most tubules. In CdCl2-treated rat testes (c), p-FAK-Tyr407was no longer detectable at the BTB (see ‘open’ white arrowheads), which is the magnified image of the ‘white’ boxed area in the right column inc, and p-FAK-Tyr407was also considerably diminished. p-FAK-Tyr407appeared as vesicle-like structures near the tubule lumen in rats after treatment (and also in CdCl2-treated rats), representing cytoplasmic droplets from p-FAK-Tyr407-positive materials engulfed by Sertoli cells23. Scale bar=50 μm in (a–c), which applies to all micrographs in the first three columns in (a–c); scale bar in the ‘yellow’ boxed micrograph=20 μm, which applies to all ‘blue’ and ‘green’ boxed micrographs ina,b; scale bar in the last micrograph inc=80 μm. DAPI, 4',6-diamidino-2-phenylindole. Figure 7: Laminin F5-peptide disrupts BTB and spermatid adhesion via p-FAK-Tyr 407 . Testes received vehicle (control) at time 0 ( a ) versus synthetic F5-peptide at 80 μg per testis (~10 μM), and terminated at 3 days, and 1, 2 and 4 weeks ( b ), and positive control where rats were treated with CdCl 2 (5 mg kg −1 body weight, intraperitoneal, for 5 days) ( c ). In control testes, p-FAK-Tyr 407 was localized near the basement membrane consistent with its localization at the BTB (see ‘yellow’ boxed area in the micrograph on the left, which was magnified in the right panel (top) in each row with the relative BTB location annotated by the ‘broken white-line’); p-FAK-Tyr 407 was also found in the adluminal compartment, restricted almost exclusively to the concave side of the spermatid head at the apical ES (see ‘blue’ and ‘green’ boxed areas in the micrograph on the third column, which were magnified in the right panel (bottom) in each row). Following F5 peptide treatment, p-FAK-Tyr 407 was downregulated and mis-localized at the BTB, as it no longer restricted to the BTB, but diffused away (see ‘white’ bracket on the top right panel of each column in treatment groups versus control rats, which was widened over time in treatment groups). p-FAK-Tyr 407 was also downregulated and its localization at the apical ES also shifted from the concave to cover the convex side of the spermatid head by 3-day, and p-FAK-Tyr 407 no longer associated with the apical ES in most elongated spermatids by 1 and 2 weeks, and by 4 weeks as elongated spermatids were not found in most tubules. In CdCl 2 -treated rat testes ( c ), p-FAK-Tyr 407 was no longer detectable at the BTB (see ‘open’ white arrowheads), which is the magnified image of the ‘white’ boxed area in the right column in c , and p-FAK-Tyr 407 was also considerably diminished. p-FAK-Tyr 407 appeared as vesicle-like structures near the tubule lumen in rats after treatment (and also in CdCl 2 -treated rats), representing cytoplasmic droplets from p-FAK-Tyr 407 -positive materials engulfed by Sertoli cells [23] . Scale bar=50 μm in ( a – c ), which applies to all micrographs in the first three columns in ( a – c ); scale bar in the ‘yellow’ boxed micrograph=20 μm, which applies to all ‘blue’ and ‘green’ boxed micrographs in a , b ; scale bar in the last micrograph in c =80 μm. DAPI, 4',6-diamidino-2-phenylindole. Full size image F5 peptide perturbs cell adhesion via F-actin organization It was recently shown that p-FAK-Tyr 407 mediated its effects via Arp-3 of the Arp-2/3-N-WASP complex, modulating branched actin polymerization, causing F-actin reorganization in Sertoli cells, thereby regulating cell adhesion at the BTB in the rat testis [23] . As overexpression of the F5 fragment in the Sertoli cell epithelium ( Fig. 2a ) or administration of F5 peptide into the testis ( Fig. 4e ) also downregulated and/or induced mis-localization of p-FAK-Tyr 407 ( Fig. 7 ), we next investigated changes in the distribution of actin filament bundles in the seminiferous epithelium by staining F-actin using phalloidin-FITC. Although the total actin determined by immunoblotting in both treatment groups versus controls were similar (see Fig. 4e ), significant changes in the distribution and/or localization of F-actin at the apical ES and the BTB in the seminiferous epithelium following F5 peptide treatment were detected ( Fig. 8 ). Specifically, actin filaments (that is, F-actin) were no longer tightly packed at the BTB, but they were mis-localized, moving away from the Sertoli cell–cell interface at the BTB ( Fig. 8 ). Because of the peptide-induced depletion of elongated/elongating spermatids from the epithelium, F-actin at the apical ES site was also mis-localized ( Fig. 8 ). These changes in F-actin organization thus contribute to an alteration of occludin localization at the BTB (see Fig. 6 ), destabilizing cell adhesion at the Sertoli–Sertoli cell interface, leading to BTB disruption ( Fig. 4c–e ), and premature release of spermatids ( Fig. 5a–e , Supplementary Fig. S2 ) from the epithelium. 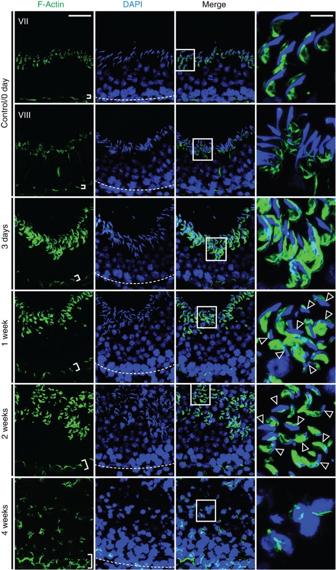Figure 8: Laminin F5 peptide induces spermatid loss via changes in F-actin distribution. Rat testes received synthetic F5 peptide at 80 μg per testis (~10 μM) at time 0, and terminated at 3 days, and 1, 2 and 4 weeks versus control (normal rats). Frozen sections were used to visualize the distribution of F-actin in the seminiferous epithelium. Relative location of the BTB was annotated by the ‘white’ broken line in the panel stained for cell nuclei with 4',6-diamidino-2-phenylindole (DAPI). Actin filaments were most abundant at the BTB and the apical ES at the Sertoli-spermatid interface as shown in a stage VII and VIII tubule in control rats at time 0. By 3 days, 1, 2 and 4 weeks after F5 peptide treatment, in tubules of stage ~VII-VIII, actin filaments were redistributed, progressively moving away from the BTB site (see the ‘white’ brackets that illustrate the relatively ‘tightly’ packed actin filaments, such as those found in controls, were ‘unbundled’ and the ‘white’ brackets were widened in treated rat testes). Although F-actin was also restricted to the apical ES at these time points, actin filaments were no longer tightly restricted to the Sertoli–spermatid interface at the apical ES as seen in control testes (see ‘magnified’ images in the last column of the ‘boxed’ areas in the third column). Moreover, actin filaments were no longer restricted to the elongated spermatids as shown in control testes, but were also found in early elongating spermatids (see ‘open’ arrowheads). This mis-localization of the F-actin network at the apical ES no longer supported spermatid adhesion, causing premature ‘spermiation’. Scale bar=50 μm in the micrograph in the first column, which applies to all micrographs in the first three columns, scale bar=20 μm in the micrograph in the fourth column, which applies to all micrographs in this column. Figure 8: Laminin F5 peptide induces spermatid loss via changes in F-actin distribution. Rat testes received synthetic F5 peptide at 80 μg per testis (~10 μM) at time 0, and terminated at 3 days, and 1, 2 and 4 weeks versus control (normal rats). Frozen sections were used to visualize the distribution of F-actin in the seminiferous epithelium. Relative location of the BTB was annotated by the ‘white’ broken line in the panel stained for cell nuclei with 4',6-diamidino-2-phenylindole (DAPI). Actin filaments were most abundant at the BTB and the apical ES at the Sertoli-spermatid interface as shown in a stage VII and VIII tubule in control rats at time 0. By 3 days, 1, 2 and 4 weeks after F5 peptide treatment, in tubules of stage ~VII-VIII, actin filaments were redistributed, progressively moving away from the BTB site (see the ‘white’ brackets that illustrate the relatively ‘tightly’ packed actin filaments, such as those found in controls, were ‘unbundled’ and the ‘white’ brackets were widened in treated rat testes). Although F-actin was also restricted to the apical ES at these time points, actin filaments were no longer tightly restricted to the Sertoli–spermatid interface at the apical ES as seen in control testes (see ‘magnified’ images in the last column of the ‘boxed’ areas in the third column). Moreover, actin filaments were no longer restricted to the elongated spermatids as shown in control testes, but were also found in early elongating spermatids (see ‘open’ arrowheads). This mis-localization of the F-actin network at the apical ES no longer supported spermatid adhesion, causing premature ‘spermiation’. Scale bar=50 μm in the micrograph in the first column, which applies to all micrographs in the first three columns, scale bar=20 μm in the micrograph in the fourth column, which applies to all micrographs in this column. Full size image Herein, we have identified the biologically active domain in laminin-γ3 DIV of the laminin-γ3 chain from laminin-333 residing at the apical ES, which is comprised of a stretch of 50 amino-acid residues designated F5 peptide, and a synthetic F5 peptide was found to be capable of reversibly perturbing the BTB in vivo , leading to germ cell exfoliation from the seminiferous epithelium of adult rat testes. These effects were found to be mediated by perturbing the restrictive spatiotemporal expression and/or localization of p-FAK-Tyr 407 , which, in turn, affects the distribution of F-actin at the apical and basal ES in the epithelium. These findings illustrate that a disruption of the apical ES-BTB-basement membrane functional axis can be a novel approach to disrupt spermatogenesis. Other studies in the field also support the concept that biologically active collagen fragments can be used to manipulate the TJ-permeability barrier function in blood–tissue barriers [13] , [38] . For instance, although a 20 kDa fragment derived from collagen XVIII, known as endostatin, was ineffective per se to modulate the TJ-permeability barrier of retinal microvascular endothelial cells (RMEC), it was found to induce a significant increase of occludin expression at the RMEC TJ barrier [39] . Furthermore, endostatin was capable of blocking the vascular endothelial growth factor-mediated TJ-barrier disruption in RMEC by altering the phosphorylation status of occludin at the blood–retinal barrier [39] via an activation of ERK1/ERK2 and p38 MAPK [40] . In the testis, collagens such as collagen α3(IV) chains are abundant at the basement membrane, which is a modified form of the extracellular matrix [2] , [38] . In addition, other studies have also illustrated that a degradation of laminin 332 by plasmin [41] was found to impair keratinocyte adhesion and the assembly of basement membrane at the dermal–epidermal junction. Also, a deletion of collagen XVIII (in Col18α1 −/− mice) or an overexpression of its endostatin domain) was found to accelerate or delay cutaneous wound healing, respectively [42] . Collectively, these data thus indicate unequivocally that collagen and/or laminin fragments, some of these are biologically active peptides, can be generated during in vivo cellular processing to modulate diversified cellular functions. In short, F5 peptide generated at the apical ES during spermiation via cleavage of the laminin-γ3 chain by MMP2 near the apical region of the Sertoli cell epithelium can exert its effects near the basal region of the epithelium to induce BTB restructuring, mediated by changes in the expression and/or localization of p-FAK-Tyr 407 , to be followed by F-actin distribution and/or localization. Even though the synthetic F5 peptide disrupts the BTB integrity in vivo , the possibility of developing antisperm antibodies in these rats is unlikely because virtually all the advanced germ cells, such as post-meiotic spermatids, were depleted from the epithelium at the time of BTB disruption, and the disrupted BTB was ‘resealed’ when spermatogenesis re-initiated. As laminin chains at the apical ES are restricted to elongating/elongated spermatids, a question arises regarding the signalling mechanism(s) by which laminin fragment(s) perturbs cell adhesion at the apical and basal ES, as these biological fragments are found outside the Sertoli cell in the seminiferous epithelium in vivo . Thus, is this an ‘outside–in’ signalling analogous to biologically active collagen fragments that were found to induce integrin clustering in other cell epithelia [38] , [43] ? Our earlier studies have shown that besides laminin-γ3 chain, laminin-β3 chain also possesses biological activity in its domain I [15] . Thus, we prepared two cDNA constructs based on domain I of laminin-β3 chain that did or did not contain the signal peptide for their transient expression in Sertoli cells in vitro ( Supplementary Fig. S4 ) and to test their effects on the Sertoli cell TJ-permeability barrier function ( Supplementary Fig. S5 ). Interestingly, both constructs were capable of perturbing the Sertoli cell TJ-barrier function by downregulating occludin expression, illustrating these biologically active fragments were active by inducing either ‘outside–in’ or ‘inside–out’ signalling ( Supplementary Fig. S5 ). However, more work is needed to define the detailed molecular mechanism by which laminin fragments, such as F5 fragment, exert their effects via the ‘outside–in’ or the "inside-out" signalling, including the identification of the involved receptor(s) in Sertoli cells. It is noted that overexpression of F5 peptide in Sertoli cells with an established functional TJ barrier or direct administration of synthetic F5 peptide into the rat testis were both found to perturb cell adhesion at the Sertoli cell BTB, perturbing Sertoli cell TJ-permeability barrier function in vitro and in vivo , as well as spermatid adhesion at the apical ES in vivo . However, the efficacy of overexpression was limited to ~20% (see Supplementary Methods ), whereas the efficacy via local administration of F5 peptide in the testis was at ~40%. Thus, an improved delivery methodology remains to be developed, such as involving the use of protein transduction domain [44] , [45] , genetic engineered F5 peptide into an follicle stimulating hormone (FSH) mutant [46] , or nanoparticle-based F5-petide [47] , [48] . In summary, we have identified the biologically active domain of laminin-γ3 domain IV, which is highly effective in perturbing the Sertoli cell TJ-permeability barrier function both in vitro and in vivo , mediating its effects via p-FAK-Tyr 407 , affecting the localization and/or distribution of TJ integral membrane proteins (for example, occludin) at the site via changes in the organization and/or distribution of F-actin at the Sertoli–Sertoli and Sertoli–spermatid adhesion sites. It was found that the administration of the F5 peptide in the testis that perturbs the apical ES–BTB–basement axis also leads to germ cell exfoliation and impairs spermatogenesis. Additional studies are now warranted to investigate if this peptide can be developed into a male contraceptive. Several other questions also remain to be addressed in future studies. For instance, do other epithelial cells, such as MDCK cells, that establish apical junctions respond to F5 peptide similar to Sertoli cells? Would the F5 peptide remain in the Sertoli cell, or be confined in cell cytosol or in membranous compartments if it were overexpressed? If peptide fragments are released at spermiation at the apical region of the Sertoli cell, they presumably exert their effects via receptors (such as integrins at the apical ES in Sertoli cells [10] ) and/or signalling molecules (for example, p-FAK-Tyr 397 or -Tyr 407 ) [23] at the apical ES to generate a signalling cascade that leads to changes in basal junctions at the BTB. How would administering the peptide basally to Sertoli cells in vivo have any effect, as receptors would presumably be concentrated above the BTB? We expect that some of these questions will be addressed in the near future. Animals Male Sprague–Dawley rats (20-day-old pups; and adult males at ~250–300 g body weight) were purchased from Charles River Laboratories (Kingston, NY). The use of animals was approved by the Rockefeller University Institutional Animal Care and Use Committee with Protocol Numbers 09016 and 12506. Overexpression of laminin fragments or the FAK mutant Laminin fragments F1–F8 corresponding to different stretches of sequence of laminin-γ3 domain IV chain ( Fig. 1 , Supplementary Fig. S1 ) were cloned into pCIneo mammalian expression vector (Promega) at sites between Xho I and Sal I by using specific primers ( Supplementary Table S1 ). The authenticity of these clones was confirmed by direct nucleotide sequencing at Genewiz Inc (South Plainfield, NJ). p-FAK phosphomimetic mutant FAK Y407E was generated using a full-length rat FAK clone prepared in our laboratory by site-directed mutagenesis as earlier described [23] , and it was also cloned into the Mlu I/ Xba I sites of the pCIneo vector. Before their use, plasmid DNA was purified using the HiSpeed Plasmid Midi Kit (Qiagen). On day 3, after a functional Sertoli cell TJ-permeability barrier was established, cells at 0.5 × 10 6 cells cm −2 in 12-well dishes (with 3-ml F12/DMEM per well) or at 1.2 × 10 6 cells cm −2 in bicameral units placed in 24-well dishes (with 0.5 ml F12/DMEM each in the apical and basal compartment) were transfected with either 1 or 0.5 μg plasmid DNA by using Effectene Transfection Reagent (Qiagen) at a ratio of 15 μl to 1 μg DNA. Transfection mixture was removed 24 h thereafter and replaced with fresh F12/DMEM. RNA and protein lysates were obtained from these cultures 2 and 3 days thereafter, respectively. The TJ-permeability barrier after transient expression of laminin-γ3 domain IV fragments versus pCIneo vector alone was also assessed by transepithelial electrical resistance (TER) measurement across the Sertoli cell epithelium as described earlier [49] . Treatment of rat testes with synthetic F5 peptide Adult rats weighing ~250–275 g body weight ( n =~5–6 rats per time point in both treatment and control groups) received a single dose of the F5 synthetic peptide (relative molecular mass at 5,630.36) at either 80 μg (~10 μM) or 320 μg (~40 μM) per testis (testis weight at ~1.6 g, assuming a volume of ~1.6 ml) via direct intratesticular injection using a 28-gauge needle in a final injection volume of ~200 μl (in 0.9% saline) as described earlier [31] , [50] . These concentrations of synthetic F5 peptide were selected based on results of the in vitro study in which 50 μg ml −1 (~10 μM) was found to consistently and reversibly perturb the Sertoli cell TJ-permeability barrier. In some experiments, the right testis received the synthetic F5-peptide and the left testis received vehicle alone (saline alone without synthetic peptide) to serve as a negative control. Rats were terminated on day 3, and 1, 2 and 4 weeks thereafter. Rats were euthanized by CO 2 asphyxiation, and testes were removed. In selected experiments, testes were either fixed in Bouin’s fixative to be used for paraffin embedding and sectioning for hematoxylin and eosin staining for histological analysis as described [27] , or snap-frozen in liquid nitrogen and stored at −80 °C until used to obtain frozen sections for immunohistochemistry or immunoblotting. In some experiments, rats at specified time points were subjected to an in vivo assay to assess BTB integrity. Selected rats were treated with the 22-amino acid MTMR2 peptide at 200 μg per testis (~50 μM) and terminated at 1, 4 and 8 weeks for histological analysis ( n =3 rats per time point), and no alterations in the status of spermatogenesis were noted, consistent with an earlier report [31] . Thus, these rats were not used for subsequent BTB integrity assays. Other Materials and Methods pertinent to this report, such as primary Sertoli cell cultures, preparation of cDNA constructs to assess ‘inside–out’ and ‘outside–in’ signalling, BTB integrity assay, dual-labeled immunofluorescence analysis, immunohistochemistry, F-actin staining, immunoblot analysis and statistical analyses can be found in Supplementary Materials and Methods . How to cite this article: Su, L. et al. A peptide derived from laminin-γ3 reversibly impairs spermatogenesis in rats. Nat. Commun. 3:1185 doi: 10.1038/2171 (2012).